Activation ofXistby an evolutionarily conserved function of KDM5C demethylase XX female and XY male therian mammals equalize X-linked gene expression through the mitotically-stable transcriptional inactivation of one of the two X chromosomes in female somatic cells. Here, we describe an essential function of the X-linked homolog of an ancestral X-Y gene pair, Kdm5c - Kdm5d , in the expression of Xist lncRNA, which is required for stable X-inactivation. Ablation of Kdm5c function in females results in a significant reduction in Xist RNA expression. Kdm5c encodes a demethylase that enhances Xist expression by converting histone H3K4me2/3 modifications into H3K4me1. Ectopic expression of mouse and human KDM5C , but not the Y-linked homolog KDM5D , induces Xist in male mouse embryonic stem cells (mESCs). Similarly, marsupial (opossum) Kdm5c but not Kdm5d also upregulates Xist in male mESCs, despite marsupials lacking Xist , suggesting that the KDM5C function that activates Xist in eutherians is strongly conserved and predates the divergence of eutherian and metatherian mammals. In support, prototherian (platypus) Kdm5c also induces Xist in male mESCs. Together, our data suggest that eutherian mammals co-opted the ancestral demethylase KDM5C during sex chromosome evolution to upregulate Xist for the female-specific induction of X-inactivation. X and Y chromosomes in therian mammals evolved from an ordinary pair of normally recombining autosomes [1] , [2] , [3] . As the Y chromosome formed, its ability to recombine with the X chromosome decreased incrementally and it lost much of its gene content [4] . Consequent to the loss of Y-linked genes in males, eutherian (placental) and metatherian (marsupial) females ultimately evolved X-chromosome inactivation, which silences genes along one of the two X chromosomes, thereby equalizing X-linked gene expression between the sexes [5] . Although most X–Y homologs have been lost from the Y chromosome, some remain intact and functional. Moreover, the X-linked homologs of ancestral Y-linked genes that are broadly expressed almost invariably escape X-inactivation [6] , [7] . Escape from inactivation is thought to ensure similar combined expression of X–Y gene pairs between the sexes and is premised upon the homologs being functionally equivalent to one another [6] , [7] . Ancestral X–Y gene pairs, however, have been separated for ~100 million years and have accumulated amino acid substitutions due to lack of recombination [6] , [7] . Escape from X-inactivation of diverged X–Y gene pairs can lead to increased expression of the X-linked homolog in females vs. males and contribute to sexually dimorphic effects [8] , [9] , including potentially in X-inactivation in females [10] , [11] . Stable X-inactivation in eutherians requires the Xist long noncoding RNA [12] , [13] , which is upregulated from and physically coats the future inactive X chromosome [14] , [15] . Xist RNA accumulation directly or indirectly recruits a suite of proteins that in turn stably silence X-linked genes [16] , [17] , [18] , [19] , [20] . How Xist RNA is preferentially upregulated in females, but not males, remains unclear [11] . Xist and all of its transcriptional regulatory elements, including both cis -acting sequences and trans -acting factors, are believed to reside within the X-inactivation center ( Xic ) region of the X chromosome [21] , [22] . The Xic is thought to be both necessary and sufficient to induce X-inactivation [21] , [23] , [24] . One model of female-specific induction of X-inactivation relies on the sensing of the X chromosome complement via the physical pairing of the two Xs in XX cells through sequences within the Xic [25] . This coupling of the X chromosomes is proposed to result in a transvection-like mechanism that induces Xist RNA in XX females but not in XY males [26] , [27] , [28] . However, deletions of all candidate Xic elements involved in X chromosome pairing fail to prevent Xist upregulation from an X chromosome in differentiating female mouse embryonic stem cells (ESCs) [10] , [29] , which stochastically silence one of their two Xs during the process of random X-inactivation [30] . Moreover, physical separation of the two X chromosomes by tethering of one or both X chromosomes in female ESCs to the nuclear lamina nevertheless led to Xist induction upon differentiation of the ESCs [31] . Another candidate mechanism underlying the female-specific induction of Xist RNA is the increased expression in XX females vs. XY males of Xic -encoded diffusible Xist activators that function in trans . The X-linked Rnf12 / Rlim gene has been proposed to encode such a dose-dependent activator of Xist [32] . When ectopically expressed in XY male ESCs, Rnf12 , which encodes an E3 ubiquitin ligase, can induce Xist in a subset of the cells [32] . Rnf12 is also required to maintain Xist RNA expression during imprinted X-inactivation in mice [33] . Imprinted X-inactivation results in the silencing exclusively of genes on the paternally-inherited X chromosome in all cells of the preimplantation mouse embryo [34] , [35] . An Rnf12 mutation on the maternally-derived X chromosome results in reduced Xist RNA expression from the paternal X chromosome in morula-stage female mouse embryos [33] . Rnf12 , however, appears to be dispensable for Xist RNA induction during random X-inactivation that characterizes the epiblast lineage, which gives rise to all the somatic cell types and germ cells in the mouse embryo [34] , [35] , [36] , [37] . Rnf12 +/− and Rnf12 −/− female mouse embryonic epiblasts and differentiating female ESCs can upregulate Xist RNA expression, which suggests that alternate factors can induce Xist RNA in a dose-dependent manner during random X-inactivation [29] , [32] , [36] , [37] . The Xic -linked Ftx and Jpx / Enox lncRNA-expressing loci have also been proposed to activate Xist expression in females [38] , [39] , [40] . However, deletions of Ftx and Jpx / Enox together with Rnf12 on an X chromosome do not abrogate Xist induction in differentiating XX female ESCs but may lead to reduced Xist expression in cis from the mutant X chromosome [29] . These results suggest that Ftx and Jpx / Enox loci do not function as dose-dependent and diffusible trans -acting activators of Xist that induce X-inactivation selectively in females [41] . Other lncRNA-expressing loci in the Xic also appear to regulate Xist in cis , but not in trans [10] , [42] . Our prior work suggested that Xist is preferentially induced in females at the onset of random X-inactivation by gene(s) that later escape X-inactivation [11] . We found that a disruption of the Xist antisense repressor Tsix ectopically induced Xist from the active Tsix -mutant X chromosome ( X Δ Tsix ) in differentiating pluripotent stem cells of both sexes in vivo and in vitro [10] , [11] . Interestingly, however, the ectopic expression of Xist RNA from the active X Δ Tsix occurred in greater numbers of differentiating X Δ Tsix X female pluripotent embryonic epiblast cells and cultured epiblast stem cells (EpiSCs) compared to X Δ Tsix Y male cells [11] . EpiSCs are primed pluripotent stem cells [43] , [44] , which capture X-inactivation shortly after it has begun [10] , [11] . Since female EpiSCs harbor an inactivated X chromosome, we hypothesized that the increased dose in X Δ Tsix X females compared to X Δ Tsix Y males of one or more genes which escape X-inactivation underlie the more robust ectopic Xist induction in differentiating X Δ Tsix X female vs. X Δ Tsix Y male EpiSCs [11] . We further postulated that the higher expression of such genes in females vs. males was also responsible for Xist expression at the onset of X-inactivation in wild-type female epiblast cells [11] . The discovery and characterization of such factor(s) promised to explain the female-specific induction of random X-inactivation. Through in vivo and in vitro experiments, we reveal a role for the evolutionarily conserved X-inactivation escapee Kdm5c , which encodes a histone H3 di- and tri-methylated lysine 4 (H3K4me2 and H3K4me3) demethylase [45] , [46] , in the dose-dependent upregulation of Xist expression in eutherian mammals. Kdm5c is required for robust Xist RNA expression in the mouse epiblast lineage We nominated the lysine demethylase KDM5C as a candidate activator of Xist for two primary reasons. First, Kdm5c is a part of an ancestral X–Y chromosomal gene pair that is conserved across therian mammals [6] , [7] . Kdm5c escapes X-inactivation in both mouse and human [47] , [48] , [49] , [50] and exhibits an X-inactivation escapee chromatin profile in opossum [51] , a marsupial species, suggesting a dose-dependent and evolutionarily conserved function. Second, hypomethylation of H3K4 is associated with Xist induction [52] , [53] . Because our prior work suggested that female EpiSCs express Xist activator(s) at a higher level than male EpiSCs [11] , we tested the relative levels of Kdm5c RNA in female vs. male EpiSCs by RT-qPCR. Kdm5c was consistently more highly expressed in female vs. male EpiSCs (Fig. 1a ). We also quantified relative Kdm5c RNA levels in female vs. male ESCs. Whereas XX EpiSCs harbor an inactivated X chromosome, XX ESCs are in a pre-X inactivated state with two active X chromosomes and undergo X-inactivation only upon differentiation [30] . Kdm5c was also more highly expressed in female ESCs than in male ESCs (Fig. 1b ). Kdm5c is therefore expressed more highly in female vs. male cells both after and prior to the initiation of X-inactivation, as we predict for an activator of Xist . Fig. 1: Lethality of Kdm5c Δ/Δ female embryos. a , b Relative quantification of Kdm5c RNA levels in wild-type XX female and XY male EpiSCs ( a ) and ESCs ( b ) by RT-qPCR. Each bar in the graph represents an individual cell line analyzed by RT-qPCR in triplicate. Data are presented as mean \(\pm\) standard deviation between technical replicates. c – f Quantification of liveborn mice ( c – e ) and recovery of embryonic day ( E ) 5.5 and 6.5 embryos ( f ). g Representative micrographs of E5.5 embryos. 13 litters were analyzed with similar results. Scale bars, 50 μm. Expression of a paternally-inherited X-Gfp transgene marks female embryonic epiblasts (Epi) but not extraembryonic ectoderm (EE) or visceral endoderm (VE) due to random X-inactivation in the epiblast lineage and imprinted X-inactivation of the paternal X-chromosome in extraembryonic lineages [60] , [61] . See also Supplementary Fig. 1a . Source data are provided as a Source Data file. Full size image To test a female-specific role for Kdm5c , we took advantage of a lox p flanked (“floxed” or “fl”) conditionally mutant Kdm5c mouse strain [54] . Upon Cre -mediated recombination, the Kdm5c fl allele generates a Kdm5c Δ allele that lacks Kdm5c exons 11 and 12 (Supplementary Fig. 1a ), which encode the enzymatic Jumonji-C (JmjC) demethylase domain and produces a barely detectable mutant protein [54] , [55] . A cross of Kdm5c fl/Δ females with Kdm5c Δ Y males produced viable Kdm5c Δ Y males but not Kdm5c Δ/Δ females (Fig. 1c ). We next crossed Kdm5c fl/Δ females harboring a Zp3-Cre transgene with Kdm5c Δ Y males. The expression of the Zp3-Cre transgene deletes floxed alleles in growing oocytes and thus ensures that the resulting embryos are depleted of any oocyte-derived KDM5C protein [56] , which may influence gene expression in the early embryo [57] . This cross also produced Kdm5c Δ Y males but no Kdm5c Δ/Δ females (Fig. 1d ). Whereas embryonic epiblast cells of post-implantation female embryos undergo random X-inactivation, extraembryonic tissues maintain imprinted X-inactivation of the paternal X-chromosome that initiates in the preimplantation embryo [34] , [40] , [57] , [58] . We compared a requirement for Kdm5c in the epiblast vs. extraembryonic ectoderm by conditionally deleting Kdm5c using a Sox2-Cre transgene that efficiently excises floxed sequences in the nascent epiblast [59] . As with the crosses that generated constitutively mutant Kdm5c Δ/Δ females (Fig. 1d ), the epiblast-specific deletion of Kdm5c resulted in the absence of liveborn Kdm5c Δ/Δ females (Fig. 1e ). To define when Kdm5c Δ/Δ females were being lost, we isolated embryonic day (E) 5.5 and E6.5 post-implantation embryos from control and test crosses. In these crosses, the sires harbored a Gfp transgene on the X chromosome ( X-Gfp ), which is only transmitted to female progeny and thus permits visual sexing of the embryos [60] , [61] . Whereas the control crosses generated the expected distribution of female and male embryos, the test cross yielded fewer E5.5 and E6.5 Kdm5c Δ/Δ female embryos compared to Kdm5c Δ Y male embryos (Fig. 1f ). Moreover, the surviving Kdm5c Δ/Δ E5.5 embryos were smaller relative to their heterozygous Kdm5c fl/Δ female and Kdm5c fl Y male littermates (Fig. 1g ). From the results shown in Fig. 1 , we surmised that the under-representation of E5.5 Kdm5c Δ/Δ embryos may be due to defective random X-inactivation, which begins in the epiblast cells between E5.0-E5.25 stage of embryogenesis [10] , [62] . We therefore isolated E5.5 embryonic epiblasts and examined Xist expression by RNA fluorescence in situ hybridization (FISH) and RT-qPCR. Compared to Kdm5c fl/fl and Kdm5c fl/Δ cells, a significant number of E5.5 Kdm5c Δ/Δ epiblast nuclei lacked large Xist RNA coats by RNA FISH (Fig. 2a ). In addition, Kdm5c Δ/Δ epiblasts showed a higher proportion of nuclei with dispersed or small Xist RNA signals (Fig. 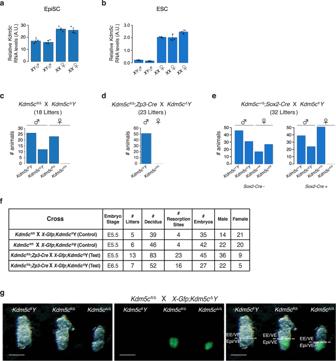Fig. 1: Lethality ofKdm5cΔ/Δfemale embryos. a,bRelative quantification ofKdm5cRNA levels in wild-typeXXfemale andXYmale EpiSCs (a) and ESCs (b) by RT-qPCR. Each bar in the graph represents an individual cell line analyzed by RT-qPCR in triplicate. Data are presented as mean\(\pm\)standard deviation between technical replicates.c–fQuantification of liveborn mice (c–e) and recovery of embryonic day (E) 5.5 and 6.5 embryos (f).gRepresentative micrographs of E5.5 embryos. 13 litters were analyzed with similar results. Scale bars, 50 μm. Expression of a paternally-inheritedX-Gfptransgene marks female embryonic epiblasts (Epi) but not extraembryonic ectoderm (EE) or visceral endoderm (VE) due to random X-inactivation in the epiblast lineage and imprinted X-inactivation of the paternal X-chromosome in extraembryonic lineages60,61. See also Supplementary Fig.1a. Source data are provided as a Source Data file. 2b and Supplementary Table 1 ). In accord with the RNA FISH data, RT-qPCR also revealed significantly reduced Xist RNA expression in E5.5 Kdm5c Δ/Δ epiblasts compared to Kdm5c fl/fl and Kdm5c fl/Δ epiblasts (Fig. 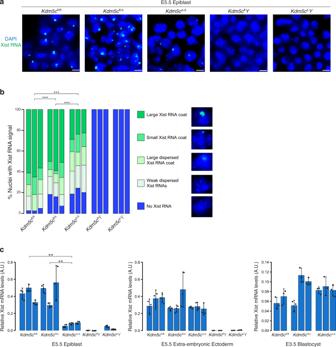Fig. 2: Reduced Xist RNA expression inKdm5cΔ/Δfemale embryos. aStrand-specific RNA FISH detection of Xist RNA in representative E5.5 embryonic epiblast cells. Nuclei are stained blue with DAPI. Scale bars, 10μm. RNA FISH analysis was performed on 3 embryos/genotype with similar results.bQuantification of Xist RNA-coated nuclei in the E5.5 epiblast cells. Number of nuclei counted in each of the three embryos/genotype:Kdm5cfl/fl,n= 36, 77, and 80;Kdm5cfl/Δ,n= 76, 68, and 55;Kdm5cΔ/Δ,n= 128, 139, and 84;Kdm5cflY,n= 150, 200, and 100;Kdm5cΔY,n= 100, 93, and 85.Pvalues, Chi-square test between female genotypes. *P≤ 0.05; **P< 0.01; ***P< 0.001. See Supplementary Table1for Welch’s two-sidedttest for all pairwise statistical comparisons.cRelative quantification of Xist RNA by RT-qPCR in E5.5 epiblasts, E5.5 extra-embryonic ectoderm, and E3.5 embryos. Each bar in the graph represents an individual E5.5 embryo fragment or E3.5 embryo analyzed by RT-qPCR in triplicate. Data are presented as mean\(\pm\)standard deviation between technical replicates.Pvalues, Welch’s two-sidedttest on ΔCt values of biological replicates. *P≤ 0.05; **P< 0.01; ***P< 0.001. Selected pairwise comparisons are shown. See Supplementary Table2for all pairwise statistical comparisons. See also Supplementary Fig.1b. Source data are provided as a Source Data file. 2c and Supplementary Table 2 ). On average, Xist RNA expression in Kdm5c Δ/Δ epiblasts was reduced by >80% compared to Kdm5c fl/fl and Kdm5c fl/Δ epiblasts. Fig. 2: Reduced Xist RNA expression in Kdm5c Δ/Δ female embryos. a Strand-specific RNA FISH detection of Xist RNA in representative E5.5 embryonic epiblast cells. Nuclei are stained blue with DAPI. Scale bars, 10μm. RNA FISH analysis was performed on 3 embryos/genotype with similar results. b Quantification of Xist RNA-coated nuclei in the E5.5 epiblast cells. Number of nuclei counted in each of the three embryos/genotype: Kdm5c fl/fl , n = 36, 77, and 80; Kdm5c fl/Δ , n = 76, 68, and 55; Kdm5c Δ/Δ , n = 128, 139, and 84; Kdm5c fl Y , n = 150, 200, and 100; Kdm5c Δ Y , n = 100, 93, and 85. P values, Chi-square test between female genotypes. * P ≤ 0.05; ** P < 0.01; *** P < 0.001. See Supplementary Table 1 for Welch’s two-sided t test for all pairwise statistical comparisons. c Relative quantification of Xist RNA by RT-qPCR in E5.5 epiblasts, E5.5 extra-embryonic ectoderm, and E3.5 embryos. Each bar in the graph represents an individual E5.5 embryo fragment or E3.5 embryo analyzed by RT-qPCR in triplicate. Data are presented as mean \(\pm\) standard deviation between technical replicates. P values, Welch’s two-sided t test on ΔCt values of biological replicates. * P ≤ 0.05; ** P < 0.01; *** P < 0.001. Selected pairwise comparisons are shown. See Supplementary Table 2 for all pairwise statistical comparisons. See also Supplementary Fig. 1b . Source data are provided as a Source Data file. Full size image To test if the deficiency in Xist RNA coating in Kdm5c Δ/Δ epiblast was due to a failure of differentiation of the pluripotent epiblast progenitor cells, we concurrently assayed Xist RNA expression by FISH and the REX1 protein by immunofluorescence (IF) (Supplementary Fig. 1b ). REX1 marks pluripotent epiblast progenitor cells and is rapidly downregulated when pluripotent cells differentiate [10] , concomitant with the onset of random X-inactivation [63] . As a control, we also conducted Xist RNA FISH and REX1 IF in E3.5 embryos, in which Rex1 is expressed in the pluripotent epiblast progenitor cells of the inner cell mass [64] . Unlike E3.5 embryos, the E5.5 control and Kdm5c Δ/Δ epiblast-enriched preparations were devoid of REX1 expression, indicating that they had undergone differentiation (Supplementary Fig. 1b ). We next tested Xist RNA expression in extraembryonic ectoderm cells of E5.5 embryos and in the preimplantation E3.5-stage embryos, both of which are subject to imprinted X-inactivation [34] , [40] , [57] , [58] . In contrast to the E5.5 epiblasts, Xist RNA levels in the three genotypes were comparable in female E5.5 extraembryonic ectoderm and E3.5 embryos (Fig. 2c and Supplementary Table 2 ). Xist RNA coating in Kdm5c Δ/Δ and Kdm5c fl/fl E3.5 embryos also appeared similar (Supplementary Fig. 1b ). Together, these data demonstrate that Kdm5c is required for robust Xist RNA expression during random but not imprinted X-inactivation. Epiblasts of surviving E5.5 Kdm5c Δ/Δ embryos appeared smaller than that of Kdm5c fl/Δ and Kdm5c fl Y littermates (Fig. 1g ). To address the possibility that reduced Xist RNA expression in Kdm5c Δ/Δ epiblast-enriched cells is a consequence of stunted development of the mutant embryos and to ensure quantitation of Xist induction in a pure population of cells of the epiblast lineage, we derived and analyzed Kdm5c fl/fl , Kdm5c fl/Δ , and Kdm5c Δ/Δ female ESCs. Differentiation of XX ESCs into epiblast-like cells (EpiLCs) results in the stochastic inactivation of one X chromosome [10] , [30] (Fig. 3a and Supplementary Fig. 2a ). As in the E5.5 embryonic epiblast cells, Kdm5c Δ/Δ EpiLCs showed fewer nuclei with large Xist RNA coats and a higher proportion of nuclei with dispersed or small Xist RNA signals compared to Kdm5c fl/fl and Kdm5c fl/Δ cells. (Fig. 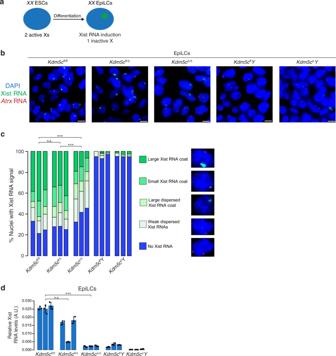Fig. 3: Reduced Xist RNA expression inKdm5cΔ/Δfemale epiblast-like cells (EpiLCs). aSchematic of induction of X-inactivation upon differentiation of ESCs into EpiLCs. See also Supplementary Fig.2a.bDetection of Xist RNA (green) by strand-specific FISH together withAtrxRNA (red) in representative EpiLCs. Scale bars, 10 μm. Three independent ESC lines were differentiated into EpiLCs/genotype with similar results.cQuantification of Xist RNA coating in EpiLCs. Xist RNA expression was quantified in five categories. Numbers of nuclei counted in EpiLCs differentiated from each of three independent ESC lines/genotype:Kdm5cfl/fl,n= 154, 122, and 113;Kdm5cfl/Δ,n= 107, 140, and 130;Kdm5cΔ/Δ,n= 145, 163, and 151;Kdm5cflY,n= 124, 230, and 111;Kdm5cΔY,n= 110, 138, and 114.Pvalues, Chi-square analysis between female genotypes. n.s. not significant; *P≤ 0.05; **P< 0.01; ***P< 0.001. See Supplementary Table3for Welch’s two-sidedttest on all pairwise statistical comparisons.dQuantification of relative Xist RNA levels by RT-qPCR in the EpiLCs. Three independent ESC lines were differentiated into EpiLCs/genotype. Each bar in graph represents an individual ESC line differentiated into EpiLCs for each genotype. Data are presented as mean\(\pm\)standard deviation between technical PCR replicates.Pvalues, Welch’s two-sidedttest on ΔCt values of biological replicates. n.s. not significant; *P≤ 0.05; **P< 0.01; ***P< 0.001. See Supplementary Table4for all pairwise statistical comparisons. See also Supplementary Fig.2b. Source data are provided as a Source Data file. 3b, c and Supplementary Table 3 ). EpiLCs of all three genotypes showed downregulation of REX1, suggesting appropriate differentiation of the mutant ESCs (Supplementary Fig. 2b ). The detection by FISH of biallelic expression of the X-linked gene Atrx demonstrates that the lack of Xist RNA coating in Kdm5c Δ/Δ EpiLCs is not due to the loss of one of the two X chromosomes in the EpiLCs (Fig. 3b ). Fig. 3: Reduced Xist RNA expression in Kdm5c Δ/Δ female epiblast-like cells (EpiLCs). a Schematic of induction of X-inactivation upon differentiation of ESCs into EpiLCs. See also Supplementary Fig. 2a . b Detection of Xist RNA (green) by strand-specific FISH together with Atrx RNA (red) in representative EpiLCs. Scale bars, 10 μm. Three independent ESC lines were differentiated into EpiLCs/genotype with similar results. c Quantification of Xist RNA coating in EpiLCs. Xist RNA expression was quantified in five categories. Numbers of nuclei counted in EpiLCs differentiated from each of three independent ESC lines/genotype: Kdm5c fl/fl , n = 154, 122, and 113; Kdm5c fl/Δ , n = 107, 140, and 130; Kdm5c Δ/Δ , n = 145, 163, and 151; Kdm5c fl Y , n = 124, 230, and 111; Kdm5c Δ Y , n = 110, 138, and 114. P values, Chi-square analysis between female genotypes. n.s. not significant; * P ≤ 0.05; ** P < 0.01; *** P < 0.001. See Supplementary Table 3 for Welch’s two-sided t test on all pairwise statistical comparisons. d Quantification of relative Xist RNA levels by RT-qPCR in the EpiLCs. Three independent ESC lines were differentiated into EpiLCs/genotype. Each bar in graph represents an individual ESC line differentiated into EpiLCs for each genotype. Data are presented as mean \(\pm\) standard deviation between technical PCR replicates. P values, Welch’s two-sided t test on ΔCt values of biological replicates. n.s. not significant; * P ≤ 0.05; ** P < 0.01; *** P < 0.001. 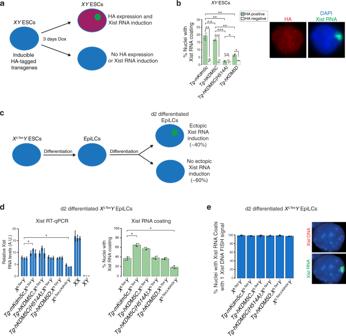Fig. 4: Ectopic KDM5C expression inducesXistin male ESCs. aSchematic of ectopic expression of HA-tagged transgenes inXYmale ESCs.bQuantification of nuclei with Xist RNA coating in transgenic (Tg)XYmale ESC lines (n= 3) expressing HA-tagged mouse KDM5C (Tg-mKdm5c;n= 292, 437, and 210); human KDM5C (Tg-hKDM5C;n= 154, 212, and 184); enzymatically inactive KDM5C (Tg-hKDM5C(H514A);45n= 292, 295, and 316); and, KDM5D (Tg-hKDM5D;n= 262, 222, and 232) proteins. Representative nuclei with IF detection of the HA epitope tag (red) coupled with FISH detection of Xist RNA (green) in theXYmale ESCs. Data are presented as mean\(\pm\)SEM.Pvalues, Welch’s two-sidedttest. n.s., not significant; *P≤ 0.05; **P< 0.01; ***P< 0.001. See Supplementary Table5for all pairwise statistical comparisons.cSchematic of ectopic Xist RNA induction in day (d) 2 differentiatedXΔTsixYmale ESCs. See also Supplementary Fig.2c, d.dQuantification of ectopic Xist RNA expression by RT-qPCR (left) and Xist RNA-coated nuclei by RNA FISH (right) in d2 differentiatedXΔTsixYEpiLCs ectopically expressing mouse KDM5C (Tg-mKdm5c;XΔTsixY); human KDM5C(Tg-hKDM5C;XΔTsixY); enzymatically inactive KDM5C (Tg-hKDM5C(H514A);XΔTsixY); KDM5D (Tg-hKDM5D;XΔTsixY); and,XΔTsixYEpiLCs lacking KDM5C (XΔTsix;ΔKdm5cY). For both the Xist RNA FISH and the Xist RT-qPCR data, three independent ESC lines/genotype were differentiated into d2 differentiated EpiLCs/genotype. For Xist RNA coating analysis,n= 100 nuclei per sample. Data are presented as mean\(\pm\)SEM. For RT-qPCR, each sample was analyzed in triplicate. Data are presented as mean\(\pm\)standard deviation between technical replicates.Pvalues, Welch’s two-sidedttest on ΔCt values of biological replicates. *P≤ 0.05; **P< 0.01; ***P< 0.001. See Supplementary Table6for all pairwise statistical comparisons.eDNA FISH following RNA FISH demonstrates the presence of one X chromosome in nuclei with ectopic Xist RNA coating in the differentiated EpiLCs.n= 100 nuclei from three independent ESC lines differentiated into EpiLCs/genotype. Data are presented as mean\(\pm\)SEM. See also Supplementary Fig.3. Source data are provided as a Source Data file. See Supplementary Table 4 for all pairwise statistical comparisons. See also Supplementary Fig. 2b . Source data are provided as a Source Data file. Full size image In agreement with the RNA FISH data, RT-qPCR also displayed significantly reduced Xist RNA levels in Kdm5c Δ/Δ EpiLCs compared to Kdm5c fl/fl EpiLCs and comparable to that found in Kdm5c fl Y and Kdm5c Δ Y male EpiLCs (Fig. 3d and Supplementary Table 4 ). On average, Xist RNA expression in Kdm5c Δ/Δ EpiLCs was reduced by >90% compared to Kdm5c fl/fl EpiLCs. Moreover, the similar expression of Xist RNA in Kdm5c Δ/Δ female and Kdm5c fl Y male EpiLCs suggests that Xist RNA induction in Kdm5c Δ/Δ female cells reflects a basal level of Xist expression. Interestingly, Kdm5c fl/Δ heterozygous EpiLCs expressed Xist at an intermediate level between Kdm5c fl/fl and Kdm5c Δ/Δ EpiLCs, suggesting a dose-dependent requirement for KDM5C in Xist RNA induction, as our hypothesis predicts. Ectopic expression of mouse and human KDM5C induces Xist RNA in male ESCs Having established that KDM5C is necessary for robust Xist RNA expression in XX female epiblast cells, we next tested the sufficiency of KDM5C in inducing Xist RNA by ectopically expressing KDM5C in XY male ESCs (Fig. 4a ). Strikingly, mouse Kdm5c ( Tg - mKdm5c ) and human KDM5C ( Tg-hKDM5C ) transgene expression resulted in induction of Xist RNA in ~15-20% of XY male ESCs (Fig. 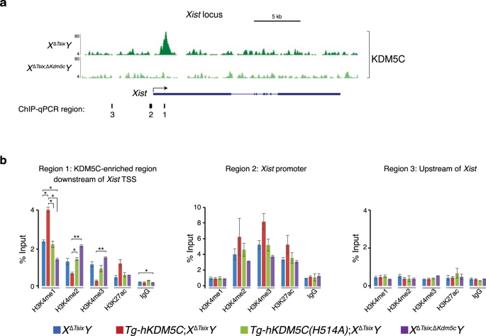Fig. 5: KDM5C upregulation ofXistexpression via putative enhancer activation. aKDM5C enrichment at theXistlocus detected by ChIP-Seq. See Supplementary Table7for ChIP-seq read quantification.bChIP-qPCR quantification of H3K4me1, H3K4me2, H3K4me3, and H3K27ac enrichment at theXistlocus. Locations of PCR amplicons are denoted beneath the browser views in (a). ChIPs were performed on day 2 differentiated EpiLCs generated from two independent ESC lines/genotype. qPCRs were performed in triplicate for each ChIP sample. Data are presented as mean\(\pm\)SEM between ChIP replicates. Selected pairwise comparisons are shown. *P≤ 0.05; **P< 0.01; ***P< 0.001, Welch’s two-sidedttests. See Supplementary Table8for all pairwise statistical comparisons. Source data are provided as a Source Data file. 4b and Supplementary Table 5 ). A transgene harboring a point mutation that abolishes the demethylase function of KDM5C ( Tg-hKDM5C(H514A) [45] , [55] ) was not able to induce Xist RNA in the XY male ESCs (Fig. 4b and Supplementary Table 5 ). Ectopic expression of the closely related homolog, KDM5D ( Tg - hKDM5D) , which maps to the Y chromosome and is itself capable of demethylating H3K4me2/3 [45] , was also able to induce Xist RNA but at a level significantly lower than mouse or human KDM5C (Fig. 4b and Supplementary Table 5 ). Thus, KDM5C and KDM5D appear to be distinct in their quantitative capabilities to activate Xist . Fig. 4: Ectopic KDM5C expression induces Xist in male ESCs. a Schematic of ectopic expression of HA-tagged transgenes in XY male ESCs. b Quantification of nuclei with Xist RNA coating in transgenic ( Tg ) XY male ESC lines ( n = 3) expressing HA-tagged mouse KDM5C ( Tg-mKdm5c ; n = 292, 437, and 210); human KDM5C ( Tg-hKDM5C ; n = 154, 212, and 184); enzymatically inactive KDM5C ( Tg-hKDM5C(H514A) ; [45] n = 292, 295, and 316); and, KDM5D ( Tg-hKDM5D ; n = 262, 222, and 232) proteins. Representative nuclei with IF detection of the HA epitope tag (red) coupled with FISH detection of Xist RNA (green) in the XY male ESCs. Data are presented as mean \(\pm\) SEM. P values, Welch’s two-sided t test. n.s., not significant; * P ≤ 0.05; ** P < 0.01; *** P < 0.001. See Supplementary Table 5 for all pairwise statistical comparisons. c Schematic of ectopic Xist RNA induction in day (d) 2 differentiated X Δ Tsix Y male ESCs. See also Supplementary Fig. 2c, d . d Quantification of ectopic Xist RNA expression by RT-qPCR (left) and Xist RNA-coated nuclei by RNA FISH (right) in d2 differentiated X Δ Tsix Y EpiLCs ectopically expressing mouse KDM5C ( Tg-mKdm5c ; X Δ Tsix Y ); human KDM5C ( Tg-hKDM5C ; X Δ Tsix Y ); enzymatically inactive KDM5C ( Tg-hKDM5C(H514A) ; X Δ Tsix Y ); KDM5D ( Tg-hKDM5D ; X Δ Tsix Y ); and, X Δ Tsix Y EpiLCs lacking KDM5C ( X Δ Tsix ;Δ Kdm5c Y ). For both the Xist RNA FISH and the Xist RT-qPCR data, three independent ESC lines/genotype were differentiated into d2 differentiated EpiLCs/genotype. For Xist RNA coating analysis, n = 100 nuclei per sample. Data are presented as mean \(\pm\) SEM. For RT-qPCR, each sample was analyzed in triplicate. Data are presented as mean \(\pm\) standard deviation between technical replicates. P values, Welch’s two-sided t test on ΔCt values of biological replicates. * P ≤ 0.05; ** P < 0.01; *** P < 0.001. 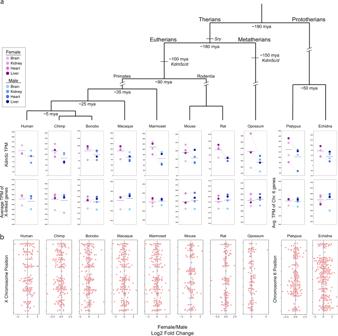Fig. 6: Phylogeny ofKdm5c/dand increased expression ofKdm5cin females vs. males in therian mammals. aInferred phylogeny ofKdm5c/dduring mammalian evolution6,7,73. Top row,Kdm5ctranscript per million (TPM) levels in four tissues, as indicated, in females vs. males for seven eutherian species, one metatherian (marsupial) species (opossum), and two prototherian (monotreme) species (platypus and echidna). Bottom row, average TPM of all X-linked genes in females vs. males in the same tissues analyzed forKdm5cexpression. Platypus and echidna TPM averages are from Chromosome (Chr) 6, where KDM5C maps in those species73. The dark gray horizontal line in all plots represents the mean of all tissues. Light gray lines connect corresponding tissue types between males and females.bDistribution of female:male expression of genes across the therian X chromosome or monotreme Chr 6. Each dot is the log2 fold change of a gene’s expression in females vs males and was calculated from the average of that gene’s TPM in the brain, heart, kidney, and liver; human plot includes expression from the brain, heart, and kidney. See Supplementary Data1–12for sequencing data from each species. See Supplementary Table 6 for all pairwise statistical comparisons. e DNA FISH following RNA FISH demonstrates the presence of one X chromosome in nuclei with ectopic Xist RNA coating in the differentiated EpiLCs. n = 100 nuclei from three independent ESC lines differentiated into EpiLCs/genotype. Data are presented as mean \(\pm\) SEM. See also Supplementary Fig. 3 . Source data are provided as a Source Data file. Full size image Dose-dependent enhancement of Xist by KDM5C To test the dose-dependent activation of Xist by KDM5C, we next took advantage of the sensitized background of X ΔTsix Y ESCs. Some but not all differentiating X ΔTsix Y male EpiLCs ectopically express Xist RNA due to a truncation of the Xist antisense repressor RNA Tsix [11] (Fig. 4c , Supplementary Fig. 2c, d , and Supplementary Fig. 3 ), which allowed us to assay changes in Xist RNA expression upon increased or decreased KDM5C expression. Compared to the parental X ΔTsix Y cells, differentiated X ΔTsix Y EpiLCs ectopically expressing mouse and human KDM5C displayed an increase in Xist RNA expression by RT-qPCR ( Tg-mKdm5c P = 0.032; Tg-hKDM5C P = 0.054; Fig. 4d and Supplementary Table 6 ). Cells ectopically expressing the enzymatically inactive KDM5C or KDM5D proteins, on the other hand, exhibited Xist RNA expression levels similar to X ΔTsix Y cells (Fig. 4d ). Reciprocally, the loss of KDM5C in X Δ Tsix ;Δ Kdm5c Y cells significantly reduced ectopic Xist RNA expression relative to X Δ Tsix Y cells ( P = 0.012; Fig. 4d and Supplementary Table 6 ). Xist RNA coating assayed by RNA FISH recapitulated the RT-qPCR data and DNA FISH confirmed the presence of a single X chromosome in these cells (Fig. 4d, e and Supplementary Table 6 ). These results are consistent with our hypothesis of a dose-dependent induction of Xist by KDM5C. Note that since Tsix is mutated in the X Δ Tsix Y EpiLCs [10] , [65] , [66] , these data rule out indirect induction of Xist by KDM5C-mediated suppression of Tsix . Xist enhancer activation by KDM5C We next sought to test if KDM5C directly activates Xist expression. We, therefore, profiled the chromatin occupancies of KDM5C and H3K4me2 by chromatin immunoprecipitation followed by sequencing (ChIP-Seq) in the differentiating X Δ Tsix Y EpiLCs examined shown in Fig. 4 . We used X ΔTsix Y male cells for ChIP analyses instead of XX female because in XX females, cellular mosaicism of X-linked gene expression due to random X-inactivation makes population measures such as ChIP-Seq and ChIP-qPCR incapable of distinguishing target molecule occupancy on the alleles of homologous X-linked genes on the inactive and active X chromosomes. In such a mosaic cell population, any incremental change in KDM5C and H3K4me2 at a given locus on the inactive X chromosome will be masked by the high levels of the mark at the homologous locus on the active X chromosome, which is enriched for the H3K4me2 [67] , [68] . We found that KDM5C is enriched ~1 kb downstream of the Xist transcriptional start site (TSS) (Fig. 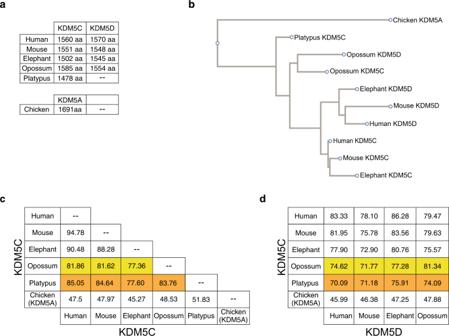Fig. 7: Divergence of KDM5C/D proteins during mammalian evolution. aAmino acid chain length of the KDM5C and KDM5D proteins.bMultiple sequence alignment phylogeny of KDM5C/KDM5D amino acid sequences using a neighbor-joining algorithm101.c,dPercent amino acid identity between therian, opossum, and platypus KDM5C proteins (c) and between KDM5C and KDM5D proteins (d). 5a and Supplementary Table 7 ). The KDM5C ChIP-Seq signal is absent in the Kdm5c -deficient X Δ Tsix ;Δ Kdm5c Y cells, demonstrating its specificity. We next questioned how KDM5C-catalyzed demethylation of H3K4me2/3, which are enriched in transcriptionally active genes, could induce Xist expression. A potential answer lay in the KDM5C-catalyzed generation of H3K4me1 upon demethylation of H3K4me2/3 [45] . H3K4me1 together with H3K27ac are enriched uniquely at enhancers [69] , [70] . We, therefore, tested H3K4me1/2/3 and H3K27ac occupancy at the KDM5C-enriched putative Xist enhancer element and two adjacent regions by ChIP-qPCR in the differentiating EpiLCs (Fig. 5b ). Fig. 5: KDM5C upregulation of Xist expression via putative enhancer activation. a KDM5C enrichment at the Xist locus detected by ChIP-Seq. See Supplementary Table 7 for ChIP-seq read quantification. b ChIP-qPCR quantification of H3K4me1, H3K4me2, H3K4me3, and H3K27ac enrichment at the Xist locus. Locations of PCR amplicons are denoted beneath the browser views in ( a ). ChIPs were performed on day 2 differentiated EpiLCs generated from two independent ESC lines/genotype. qPCRs were performed in triplicate for each ChIP sample. Data are presented as mean \(\pm\) SEM between ChIP replicates. Selected pairwise comparisons are shown. * P ≤ 0.05; ** P < 0.01; *** P < 0.001, Welch’s two-sided t tests. 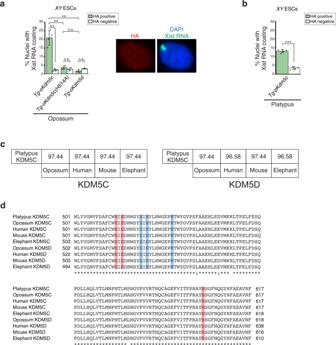Fig. 8: Opossum and platypus KDM5C activateXistin male mouse ESCs. aQuantification of nuclei with Xist RNA coating in each of three independent transgenic (Tg)XYESC lines expressing HA-tagged opossum KDM5C (Tg-oKdm5c;n= 209, 618, and 306); enzymatically inactive KDM5C protein (Tg-oKdm5c(H514A);n= 196, 206, and 193); and, KDM5D (Tg-oKdm5d;n= 803, 562, and 636). Data are presented as mean\(\pm\)SEM.Pvalues, Welch’s two-sidedttest. n.s., not significant; *P≤ 0.05; **P< 0.01; ***P< 0.001. See Supplementary Table9for all pairwise statistical comparisons.bQuantification of nuclei with Xist RNA coating in each of three independent transgenic (Tg)XYESC lines expressing HA-tagged platypus KDM5C (Tg-pKdm5c;n= 202, 178, and 525). Data are presented as mean\(\pm\)SEM.Pvalues, Welch’s two-sidedttest. ***P< 0.001. See Supplementary Table9for pairwise statistical comparisons.cPercent amino acid identity between the catalytic JmjC domain of platypus KDM5C and therian KDM5C (left) or platypus KDM5C and therian KDM5D proteins (right).dMultiple sequence alignment of the demethylase JmjC domain of KDM5C and KDM5D proteins. The predicted iron-binding and the α-ketoglutarate-binding amino acids required for the catalytic activity of KDM5C/D are shown in orange and blue55,76,102,103, respectively. Source data are provided as a Source Data file. See Supplementary Table 8 for all pairwise statistical comparisons. Source data are provided as a Source Data file. Full size image The KDM5C-enriched region downstream of the Xist TSS, Region 1, indeed displayed an enhancer-like chromatin signature of high H3K4me1 and lower H3K4me2/3 in differentiating X ΔTsix Y EpiLCs (Fig. 5b and Supplementary Table 8 ). Conversely, the Xist promoter region, Region 2, was decorated with higher H3K4me2/3 and lower H3K4me1. In Region 1, the putative Xist enhancer, ectopic expression of KDM5C but not the KDM5C H514A-mutant led to a further increase in H3K4me1 and H3K27ac along with a decrease in H3K4me2/3. In contrast, at the Xist promoter Region 2, which lacks KDM5C enrichment, we observed an increase in the active chromatin signatures H3K27ac but not H3K4me1 upon ectopic KDM5C expression (Fig. 5b and Supplementary Table 8 ). A region upstream of the Xist promoter, Region 3, did not show enrichment of the histone marks as observed in Regions 1 and 2. These data indicate that KDM5C directly promotes Xist RNA expression through the dose-dependent demethylation of H3K4me2/3 into H3K4me1 at an Xist enhancer element. An ancestral KDM5C function induces Xist The ability of human KDM5C to induce Xist in male mouse cells (Fig. 4 ) suggested that this property of KDM5C is evolutionarily conserved among eutherians. Kdm5c is an ancestral X chromosome gene that predates the eutherian and metatherian split and is intact in all therian species examined [6] , [7] . To gain insight into the extent to which the function of KDM5C is evolutionarily conserved, we first sought to test whether Kdm5c is expressed more highly in females vs. males across mammals. Kdm5c is predicted to be expressed more highly in therian females vs. males due to its likely escape from X-inactivation based on the presence of an active Y-linked Kdm5d homolog in almost all eutherians and metatherians examined [6] , [7] . To test this prediction, we measured the expression of Kdm5c in female and male tissues of seven eutherian species (human, chimp, bonobo, macaque, marmoset, rat, and mouse) and a metatherian (marsupial) species (opossum [ Monodelphis domestica ]), using prototherian (monotreme) species (platypus [ Ornithorhynchus anatinus ] and echidna [ Tachyglossus aculeatus ]) as outgroups [7] , [71] . Monotremes are the nearest extant relatives (sister taxon) of therian mammals but their X chromosomes do not undergo inactivation [6] , [7] , [72] , [73] . In the platypus and echidna, Kdm5c maps to Chromosome 6 [73] , [74] , an autosome which is thought to represent the ancestral chromosome that gave rise to the therian sex chromosomes [73] , [74] , and Kdm5d is absent. In all eight therian species, the average Kdm5c expression across the tissues examined was higher in females vs. males (1.19–1.67-fold increase in females), compared to the average expression of X-linked genes generally (0.95–1.04-fold change in females vs. males) (Fig. 6a, b and Supplementary Data 1 – 12 ). Surprisingly, Kdm5c was also more highly expressed in females vs. males in both the platypus and the echidna (1.27- and 1.60-fold increase in females compared to the 1.01- and 0.99-fold female:male ratio of average Chr 6 gene expression for platypus and echidna, respectively), which suggests that the increased Kdm5c expression in therian females may have preceded the advent of therians. Fig. 6: Phylogeny of Kdm5c/d and increased expression of Kdm5c in females vs. males in therian mammals. a Inferred phylogeny of Kdm5c/d during mammalian evolution [6] , [7] , [73] . Top row, Kdm5c transcript per million (TPM) levels in four tissues, as indicated, in females vs. males for seven eutherian species, one metatherian (marsupial) species (opossum), and two prototherian (monotreme) species (platypus and echidna). Bottom row, average TPM of all X-linked genes in females vs. males in the same tissues analyzed for Kdm5c expression. Platypus and echidna TPM averages are from Chromosome (Chr) 6, where KDM5C maps in those species [73] . The dark gray horizontal line in all plots represents the mean of all tissues. Light gray lines connect corresponding tissue types between males and females. b Distribution of female:male expression of genes across the therian X chromosome or monotreme Chr 6. Each dot is the log2 fold change of a gene’s expression in females vs males and was calculated from the average of that gene’s TPM in the brain, heart, kidney, and liver; human plot includes expression from the brain, heart, and kidney. See Supplementary Data 1 – 12 for sequencing data from each species. Full size image We next examined the size and similarity of KDM5C and KDM5D proteins between three eutherian species (mouse, human, and elephant), opossum, and platypus (Fig. 7a, b ). We found that opossum KDM5C displays a higher degree of amino acid identity to the three eutherian KDM5C proteins than to eutherian KDM5D (77.4–81.9% vs. 71.8–77.3%) (Fig. 7c, d ). Platypus KDM5C similarly exhibits greater amino acid identity to eutherian KDM5C (77.6–85.0% identity) and opossum KDM5C (83.8% identity), and lower identity to eutherian and opossum KDM5D homologs (70.1–75.9% and 74.1% identity, respectively) (Fig. 7c, d ). Fig. 7: Divergence of KDM5C/D proteins during mammalian evolution. a Amino acid chain length of the KDM5C and KDM5D proteins. b Multiple sequence alignment phylogeny of KDM5C/KDM5D amino acid sequences using a neighbor-joining algorithm [101] . c , d Percent amino acid identity between therian, opossum, and platypus KDM5C proteins ( c ) and between KDM5C and KDM5D proteins ( d ). Full size image The high level of identity among eutherian, metatherian, and prototherian KDM5C proteins prompted us to test whether Kdm5c from non-eutherian mammals could induce Xist in eutherians, e.g., mouse ESCs. Importantly, although X-inactivation occurs in all therian mammals, Xist has evolved only in eutherians and is absent in metatherians and prototherians [73] , [75] . We found that opossum KDM5C, but not KDM5D, can induce Xist RNA expression and coating in male mouse ESCs (Fig. 8a and Supplementary Table 9 ). Opossum Kdm5c containing the H514A point mutation, which is predicted to abolish the catalytic activity of KDM5C [45] , [55] , also resulted in failure to induce Xist RNA (Fig. 8a and Supplementary Table 9 ). Xist induction by both eutherian and metatherian KDM5C suggests that eutherian KDM5C has retained an ancestral therian capability which has been evolutionarily co-opted to induce Xist in eutherian mammals. Fig. 8: Opossum and platypus KDM5C activate Xist in male mouse ESCs. a Quantification of nuclei with Xist RNA coating in each of three independent transgenic ( Tg ) XY ESC lines expressing HA-tagged opossum KDM5C ( Tg-oKdm5c ; n = 209, 618, and 306); enzymatically inactive KDM5C protein ( Tg-oKdm5c(H514A) ; n = 196, 206, and 193); and, KDM5D ( Tg-oKdm5d ; n = 803, 562, and 636). Data are presented as mean \(\pm\) SEM. P values, Welch’s two-sided t test. n.s., not significant; * P ≤ 0.05; ** P < 0.01; *** P < 0.001. See Supplementary Table 9 for all pairwise statistical comparisons. b Quantification of nuclei with Xist RNA coating in each of three independent transgenic ( Tg ) XY ESC lines expressing HA-tagged platypus KDM5C ( Tg-pKdm5c ; n = 202, 178, and 525). Data are presented as mean \(\pm\) SEM. P values, Welch’s two-sided t test. *** P < 0.001. See Supplementary Table 9 for pairwise statistical comparisons. c Percent amino acid identity between the catalytic JmjC domain of platypus KDM5C and therian KDM5C (left) or platypus KDM5C and therian KDM5D proteins (right). d Multiple sequence alignment of the demethylase JmjC domain of KDM5C and KDM5D proteins. The predicted iron-binding and the α-ketoglutarate-binding amino acids required for the catalytic activity of KDM5C/D are shown in orange and blue [55] , [76] , [102] , [103] , respectively. Source data are provided as a Source Data file. Full size image Platypus KDM5C, like opossum KDM5C, is more similar to therian KDM5C than to KDM5D, suggesting that platypus Kdm5c may also harbor the ancestral biochemical KDM5C function that underlies Xist induction in eutherians. We, therefore, tested the ability of platypus KDM5C to induce Xist by expressing platypus Kdm5c in male mouse ESCs. These transgene-expressing ESCs exhibited a significantly elevated percentage of nuclei with Xist RNA coating, indicating that the platypus Kdm5c transgene can indeed induce Xist in male mouse ESCs (Fig. 8b and Supplementary Table 9 ), albeit at a slightly lower level compared to mouse, human, and opossum Kdm5c transgenes (Figs. 4 b and 8a ). This implies that the properties of KDM5C that contribute to Xist induction in eutherian females date to at least the most recent common ancestor of all extant mammalian lineages. In platypus KDM5C, the demethylating JmjC domain is 96–97% identical to the JmjC domain in therian KDM5C and KDM5D proteins, and the amino acid residues critical for co-factor binding for enzymatic activity are strictly conserved (Fig. 8c, d ) [55] , [76] , suggesting that platypus KDM5C also functions as a H3K4me2/3 demethylase. To define the amino acids that differentiate KDM5C from KDM5D, we aligned mouse, human, elephant, opossum, and platypus KDM5C and KDM5D proteins [77] (Supplementary Fig. 4a ). Among eutherians, 45 amino acids are strictly conserved across the KDM5C proteins and have no overlap with those of KDM5D, across all species (Supplementary Fig. 4b ). Among all therians (eutherians plus opossum), six amino acids are strictly conserved in KDM5C and have no overlap with KDM5D. Finally, considering all therians plus platypus, only four amino acids of KDM5C are fully conserved and fully distinct from those of therian KDM5D (prototherians lack Kdm5d ). In this study, we show that the histone H3K4me2/3 demethylase KDM5C is a primary driver of Xist RNA expression. KDM5C acts to enhance Xist RNA expression and does so in a dose- and the enzymatic-dependent manner in cells of the epiblast lineage that is subject to random X-inactivation. The biallelic and higher overall expression of Kdm5c in females vs. males links two primary steps that are thought to underlie the female-specific induction of random X-inactivation: sensing the X chromosome complement in the cell (“counting” step) and inducing expression of Xist (“initiation” step) [21] , [78] . All X chromosome sequence elements necessary and sufficient to induce X-inactivation are thought to reside within the X-inactivation center ( Xic ), which harbors the Xist locus [21] , [78] . Kdm5c , however, maps far outside of the Xic , near the telomeric end of the mouse X chromosome. Thus, the results herein suggest that elements outside of the Xic are required to induce X-inactivation through the regulation of Xist . Upon the loss of KDM5C function, Xist RNA expression in female embryonic epiblasts and EpiLCs is significantly downregulated and approaches the levels found in male samples, suggesting that KDM5C is essential for the female-specific induction of Xist ; however, residual Xist RNA expression in Kdm5c Δ/Δ epiblasts and EpiLCs suggests that other trans -acting dose-dependent factors may also contribute to Xist induction in females. Based on the results of our previous study which postulated that genes that later escape X-inactivation induce Xist at the onset of the X-inactivation process [11] , we hypothesize that, in addition to KDM5C, other dose-dependent factors encoded by X-inactivation escapees may also contribute to Xist induction. Recent work suggests that the autosomally encoded SPEN protein is required for Xist RNA induction [79] (but, see also ref. [80] ). Since Spen is an autosomal gene, its expression levels are expected to be similar between females and males. SPEN induction of Xist may thus require the increased dose of an X chromosome-encoded factor in females vs. males that, for example, directly or indirectly recruits SPEN to activate Xist in females. In support of this notion, SPEN protein binds to and is enriched within the Xist locus [79] , [81] , including in the putative enhancer element at the 5’ end of Xist where KDM5C occupancy is also enriched. Similarly, KDM5C and other escapees may recruit or potentiate the functions of other trans -acting autosomally encoded factors proposed to activate Xist [82] , [83] . X-inactivation is postulated to have evolved as a consequence of the deterioration of the Y chromosome [3] , which was once homologous to the X chromosome in the common ancestor of therian mammals [4] . By extension, the presence of active Y-linked genes is believed to have driven escape from inactivation of their X-linked homologs to adjust the dose of X–Y gene pairs between the sexes [84] . Our data instead support the notion that X–Y homologs can be functionally distinct, with the X-linked copy having evolved a female-specific function to initiate or contribute to X-inactivation. Escape from X-inactivation may therefore be evolutionarily driven in part by the requirement of the X-linked homologs in X chromosome dosage compensation. As predicted from its escape from X-inactivation, in therians we found Kdm5c is more highly expressed in the tissues of females relative to males. Unexpectedly, though, Kdm5c expression was also higher in female than male prototherians, in which Kdm5c maps to an autosome and sex-specific inactivation phenomena are unknown. It thus appears that the basis for higher levels of KDM5C in females vs. males differs between therians and prototherians, with therian females achieving it through simultaneous expression of both Kdm5c alleles via escape from X-inactivation and prototherians likely through increased expression from each Kdm5c allele in females relative to that in males. These considerations suggest that higher expression of Kdm5c in females relative to males is a fundamental mammalian characteristic that could predate the therian/prototherian divergence and the advent of X-inactivation. Of X–Y gene pairs, only Sox3/Sry , Rbmx/Rbmy , and Kdm5c/Kdm5d are conserved in all therian species examined [6] , [7] . Whereas Y-linked Sry triggers male sexual differentiation [85] and Rbmy is inferred to regulate spermatogenesis [86] , X-linked Kdm5c is required for the female-specific upregulation of Xist expression in mice. Kdm5c/d is one of only two ancestral X–Y gene pairs, along with Ube1x / y , that have diverged independently, i.e., at different times during evolution, in eutherians and metatherians [6] , [7] . The independent divergence of Kdm5d from Kdm5c in eutherians and metatherians is unlikely to be due to chance and suggests selection for the survival of the X–Y gene pair in both therian lineages [6] , [7] . Together, the increased expression of Kdm5c in females vs. males across therians suggestive of X-inactivation escape, Xist induction in eutherian cells by eutherian, metatherian, and prototherian KDM5C, and the independent differentiation of Kdm5d from Kdm5c in eutherians and metatherians suggest that an evolutionarily conserved biochemical function of KDM5C has been recruited to help induce X-inactivation selectively in females in eutherians and potentially in metatherians as well. We cautiously speculate that KDM5C may contribute to X-inactivation induction in metatherian females by dose-dependent activation of the X-linked Rsx gene, which encodes an RNA with Xist -like expression and functional properties [87] , [88] . Ethics statement This study was performed in strict accordance with the recommendations in the Guide for the Care and Use of Laboratory Animals of the National Institutes of Health. All animals were handled according to the protocols approved by the University Committee on Use and Care of Animals (UCUCA) at the University of Michigan (protocol #PRO00004007 and PRO00006455). Mice The generation of Kdm5c fl , Tsix Δ ( Tsix AA2Δ1.7 ), X-Gfp , Zp3-Cre , and JF1 strains have been described previously [54] , [56] , [60] , [66] , [89] . All mutant and transgenic strains were generated on the 129/Sv or background except for the Kdm5c fl strain, which was generated on a mixed background. The expression of the Zp3-Cre transgene deletes floxed alleles in growing oocytes and thus ensures that the resulting embryos are depleted of any oocyte-derived maternal KDM5C protein [56] , which may influence X-inactivation patterns in the early embryo. We generated mutant embryos from a cross of Kdm5c fl/Δ ; Zp3-Cre females with Kdm5c Δ/Y males harboring the X-Gfp transgene ( X-Gfp ; Kdm5c Δ/Y ). Mutant embryos were also generated from a cross of Kdm5c fl/Δ females with X-Gfp ; Kdm5c Δ/Y males. Kdm5c Δ/Δ embryos from both crosses showed similar phenotype (Fig. 1 ). The paternally transmitted X-Gfp transgene permits visual sexing of the embryos since it is only transmitted to female progeny [60] , [61] . Embryo dissections and processing Pre-, peri-, and post-implantation stage embryos were isolated essentially as described previously [65] . Briefly, E3.5 embryos were flushed from the uterine limbs in 1X PBS (Invitrogen, #14200075) containing 6 mg/ml bovine serum albumin (BSA; Invitrogen, #15260037). The zona pellucida surrounding E3.5 embryos were removed through incubation in cold Acidic Tyrode’s Solution (Sigma, #T1788), followed by neutralization through several transfers of cold M2 medium (Sigma, #M7167). GFP fluorescence conferred by the paternal transmission of the X-Gfp transgene was used to distinguish female from male embryos, since only females inherit the paternal X chromosome. Isolated embryos were either lysed for RNA isolation in 100ul of Lysis/Binding buffer (Dynabeads mRNA Direct Purification Kit, ThermoFisher, #61012) or plated onto gelatin-coated glass coverslips in 0.25× PBS with 6 mg/ml BSA for immunofluorescence (IF)/RNA fluorescence in situ hybridization (FISH) staining. For plated embryos, excess solution was aspirated, and coverslips were air-dried for 15 min. After drying, embryos were permeabilized and fixed in 50 μl solution of 0.05% Tergitol (Sigma, #NP407) and 1% paraformaldehyde (Electron Microscopy Sciences, #15710) in 1× PBS for 10 min. Excess solution was tapped off onto paper towels, and coverslips were rinsed 3× with 70% ethanol and stored in 70% ethanol at −20 °C prior to RNA FISH. For isolation of post-implantation embryos (E5.5 and E6.5), individual implantation sites were cut from the uterine limbs and decidua were removed with forceps in 1× PBS/6 mg/ml BSA. Embryos were dissected from the decidua, and the Reichert’s membranes surrounding post-implantation embryos were removed using fine forceps. The visceral endoderm layer was removed by passing the embryo through a finely pulled glass Pasteur pipet. For separation of extraembryonic and epiblast portions of embryos, fine forceps were used to physically bisect the embryos at the junction of the epiblast and extraembryonic ectoderm. The epiblast was further distinguished by GFP fluorescence conferred by the paternally transmitted X-Gfp transgene; the transgene is mosaically expressed in the epiblast due to random X-inactivation but is silenced in the extraembryonic tissues because of imprinted X-inactivation of the paternal X [60] , [61] , [90] , [91] . Extraembryonic and embryonic epiblast cells were then separately either lysed for RNA isolation in 100 µl of Lysis/Binding buffer (Dynabeads mRNA Direct Purification Kit, ThermoFisher, #61012) or plated in 0.25× PBS with 6 mg/ml BSA onto gelatinized coverslips for IF/RNA FISH staining. Samples plated for IF/RNA FISH were fixed, permeabilized, and stored as described for E3.5 embryos. Derivation and culture of embryonic stem cell (ESC) lines ESC lines were derived as previously described [30] , [92] . Briefly, individual E3.5 blastocyst are collected and plated on MEF cells in ESC derivation medium (Knockout DMEM (GIBCO, #10829-018), 20% knockout serum replacement (KSR; GIBCO, #A1099201), 2 mM l -glutamine (GIBCO, #25030), 1× nonessential amino acids (GIBCO, #11140-050), 1× penicillin–streptomycin (Gibco#15070-063), and 0.1 mM 2-mercaptoethanol (Sigma, #M7522) supplemented with 3 µM GSK3 inhibitor CHIR99021 (Stemgent#04-0004), 1 µM MEK inhibitor PD0325901 (Stemgent#04-0006), 1000 units/mL LIF (Millipore#ESG1106)) and cultured for 4–5 days. Then, individual blastocyst outgrowth is dissociated and cultured in 96 well containing MEF feeders. Mouse ESC colonies will be evident over the next 2–3 days. ESCs were cultured on mouse embryonic fibroblasts (MEFs) in knockout DMEM (GIBCO, #10829-018) with 15% knockout serum replacement (GIBCO, #A1099201), 5% ES cell qualified FBS (GIBCO, #10439024), 2 mM l -glutamine (GIBCO, #25030), 0.1 mM 2-mercaptoethanol (Sigma, #M7522), 1× nonessential amino acids (GIBCO, #11140-050), supplemented with 1000 units/ml LIF (Millipore #ESG1106). For IF and/or RNA FISH, the cells were cultured on sterilized, gelatinized coverslips. The cells were permeabilized through sequential treatment with ice-cold cytoskeletal extraction buffer (CSK:100 mM NaCl, 300 mM sucrose, 3 mM MgCl 2 , and 10 mM PIPES buffer, pH 6. 8) for 30 s, ice-cold CSK buffer containing 0.4% Triton X-100 (Fisher Scientific, #EP151) for 30 s, followed with ice-cold CSK for 30 s. After permeabilization, cells were fixed by incubation in 4% paraformaldehyde for 10 min. Cells were then rinsed 3× in 70% ethanol and stored in 70% ethanol at −20 °C prior to IF and/or RNA FISH. See Supplementary Data 13 for descriptions of all cell lines used in this study. Differentiation of ESCs into epiblast-like cells (EpiLCs) ESCs were differentiated into EpiLCs as described [30] . To convert ESC to EpiLC, ESC lines were grown in 2i culture conditions (N2B27 medium [50% DMEM/F12 (GIBCO, #11330-032), 50% neurobasal media (GIBCO, #21103-049), 2 mM l -glutamine (GIBCO, #25030), 0.1 mM 2-mercaptoethanol (Sigma, #M7522), N2 supplement (Invitrogen #17502048), B27 supplement (Invitrogen #17504-044)], supplemented with 3 μM GSK3 inhibitor CHIR99021 (Stemgent #04-0004), 1 μM MEK inhibitor PD0325901 (Stemgent #04-0006), and 1000 units/ml LIF (Millipore #ESG1106)) in gelatin-coated tissue culture dishes for four passages [93] , [94] . Following the four passages, cells were cultured in N2B27 medium supplemented with 10 ng/ml FGF2 (R&D Systems, #233-FB-025) and 20 ng/ml Activin A (R&D Systems, #338-AC-005) in fibronectin (15 μg/ml) (Sigma #F1141)-coated tissue culture dishes for 48 hrs. For X ΔTsix Y cells, after EpiLC conversion the cells were further differentiated by continuing culture in N2B27 medium without FGF2 and Activin A for an additional 48 h. For IF and/or RNA FISH, cells were permeabilized, fixed, and CSK processed as described above for ESCs. See Supplementary Data 13 for descriptions of all cell lines used in this study. Derivation and culture of epiblast stem cell (EpiSC) lines EpiSCs were derived as described [30] from E3.5 or E5.5 embryos. For the derivation of the EpiSC lines, whole E3.5 embryos or E5.5 epiblast layers were plated on MEF cells in EpiSC medium (Knockout DMEM (GIBCO, #10829-018) supplemented with 20% knockout serum replacement (KSR; GIBCO, #A1099201), 2 mM l -glutamine (GIBCO, #25030), 1× nonessential amino acids (GIBCO, #11140-050), and 0.1 mM 2-mercaptoethanol (Sigma, #M7522), 10 ng/ml FGF2 (R&D Systems, #233-FB-025)) and cultured for 3–4 days to form a large EpiSC colony. EpiSC colonies were then manually dissociated into small clusters using a glass needle and plated into 1.9-cm 2 wells containing MEF feeders in EpiSC medium. EpiSCs were passaged every third day using 1.5 mg/ml collagenase type IV (GIBCO, #17104-019) with pipetting into small clumps. See Supplementary Data 13 for descriptions of all cell lines used in this study. RNA fluorescence in situ hybridization (FISH) RNA FISH with double-stranded (ds) and strand-specific (ss) probes was performed as previously described [90] , [95] . The dsRNA FISH probes were made by randomly priming DNA templates using BioPrime DNA Labeling System (Invitrogen, #18094011). The ssRNA FISH probes were made using the Invitrogen MAXIscript Kit (Invitrogen, #AM1326). ss Xist probes were generated from templates as previously described [65] , [96] . Probes were labeled with Fluorescein-12-dUTP or -UTP (Invitrogen) or Cy3-dCTP or –CTP (GE Healthcare). Labeled probes from multiple templates were precipitated in a 0.3-M sodium acetate solution (Teknova, #S0298) (for dsRNA FISH probe) and 0.5-M ammonium acetate solution (for strand-specific RNA FISH probe) along with 300 μg of yeast tRNA (Invitrogen, #15401-029) and 150 μg of sheared, boiled salmon sperm DNA (Invitrogen, #15632-011). The solution was then spun at 21,130 rcf for 20 min at 4 °C. The pellet was washed consecutively with 70% ethanol and 100% ethanol. The pellet was dried and re-suspended in deionized formamide (ISC Bioexpress, #0606). The probe was denatured by incubating at 90 °C for 10 min followed by an immediate 5 min incubation on ice. A 2× hybridization solution consisting of 4× SSC, 20% Dextran sulfate (Millipore, #S4030), and 2.5 mg/ml purified BSA (New England Biolabs, #B9001S) was added to the denatured solution. All probes were stored at −20 °C until use. For analysis of Xist RNA coating in XY male cells that ectopically express various Kdm5c/d transgenes (Figs. 4a and 8a, b ), Xist RNA FISH was performed with a dsRNA FISH probe as well as ssRNA FISH probe. Results with both probes were concordant and were combined for the quantification. Cells or embryo fragments mounted on coverslips were dehydrated through 2 min incubations in 70%, 85%, 95%, and 100% ethanol solutions and subsequently air-dried. The coverslips were then hybridized to the probe overnight in a humid chamber at 37 °C. The samples were then washed 3× for 7 min each while shaking at 39 °C with 2XSSC/50% formamide, 3× with 2× SSC, and 2x with 1× SSC. A 1:250,000 dilution of DAPI (Invitrogen, #D21490) was added to the third 2× SSC wash. Coverslips were then mounted on slides in Vectashield (Vector Labs, #H-1000). DNA FISH DNA FISH probes were prepared as described for double-stranded RNA FISH probes [11] , [95] . The BAC template used for Xist DNA FISH is RP24-287F13 (Children’s Hospital of Oakland Research Institute). After RNA FISH, cells were washed with 1× PBS three times and then incubated in PBS for 5 min at room temperature. The cells were then re-fixed with 1% (wt/vol) PFA containing 0.5% (vol/vol) Tergitol and 0.5% (vol/vol) Triton X-100 for 10 min at room temperature. The cells were next dehydrated through an ethanol series (70%, 85%, and 100% ethanol, 2 min each) and air-dried for 15 min. The cells were then treated with RNase A (1.25 μg/μl) at 37 °C for 30 min. The cells were again dehydrated through the ethanol series as described above. The samples were then denatured in a prewarmed solution of 70% formamide in 2× SSC on a glass slide stationed on top of a heat block set at 95 °C for 11 min followed immediately by dehydration through a −20 °C-chilled ethanol series (70%, 85%, 95%, and 100% ethanol, 2 min each). The cells were then air-dried for 15 min followed by probe hybridization overnight at 37 °C. The following day, the samples were washed twice with prewarmed 50% formamide/2× SSC solution at 39 °C and 2× with 2× SSC, 7 min each. Immunofluorescence (IF) Cells mounted on glass coverslips were washed 3X in PBS for 3 min each while shaking. Coverslips were then incubated in blocking buffer consisting of 0.5 mg/ml BSA (New England Biolabs, #B9001S), 50 μg/ml yeast tRNA (Invitrogen, #15401-029), 80 units/ml RNAseOUT (Invitrogen, #10777-019), and 0.2% Tween 20 (Fisher, #BP337-100) in 1× PBS in a humid chamber for 30 min at 37 °C. The samples were next incubated with primary antibody diluted in blocking buffer for 1–3 h in the humid chamber at 37 °C. Anti-REX1 antibody (Thermo Scientific, #PA5-27567) was used at 1:150 dilution and anti-HA antibody (Cell Signaling, #C29F4) was used at 1:800 dilution. The samples were then washed 3× in PBS/0.2% Tween 20 for 3 min each while shaking. After a 5 min incubation in blocking buffer at 37 °C in the humid chamber, the samples were incubated in blocking buffer containing a 1:300 dilution of fluorescently conjugated secondary antibody (Invitrogen, Alexa Fluor 555, #A31572 for HA antibody; Alexa Fluor 647, #A31573 for REX1 antibody) for 30 min in the humid chamber at 37 °C, followed by three washes in PBS/0.2% Tween 20 while shaking for 3 min each. The samples were then processed for RNA FISH. RT-qPCR Total RNA from cells was isolated from TRIzol (Life Technologies, #15596-018) according to the manufacturer’s instructions. mRNA from embryos was purified using Dynabeads mRNA direct Purification Kit (ThermoFisher, #61012) according to the manufacturer’s instructions. RT-qPCR was performed using SYBR Green-based relative quantification method on an Eppendorf Realplex Mastercycler (software version 2.2.0.84). The housekeeping gene Gapdh was used as an internal control for data normalization. Control reactions lacking reverse transcriptase for each sample were also performed to rule out genomic DNA contamination. RT-qPCR was carried out using the SYBR Green PCR Mastermix (Kapa Sybr Fasr One-Step Universal kit #KK4651 and/or Luna Universal One-Step RT-qPCR Kit #E3005L). The following primers were used for RT-qPCR: Kdm5c : forward TTTGGCAGCGGTTTCCCTGTCAGT, reverse AAGACCATTCCCACATACAGCC; Rex1 : forward CCAGGTTCTGGAAGCGAGTT, reverse GCTTGAGGACACTCCAGCAT; RT-qPCR of Xist on XY male EpiSCs, XX female EpiSCs, and Tsix -mutant XY male EpiLCs: forward CAAGAAGAAGGATTGCCTGGATTT, reverse GCGAGGACTTGAAGAGAAGTTCTG. RT-qPCR of Xist on all other samples: forward CTCCCAGCATTACTGAGAAATG, reverse CCAGGCAATCCTTCTTCTTGAG. Gapdh: forward TGTGTCCGTCGTGGATCTGA, reverse CCTGCTTCACCACCTTCTTGA. P values for all RT-qPCR results were calculated using Welch’s two-sample t tests. RT-qPCR data is presented for each biological replicate. Error bars represent the standard deviation between technical replicates of multiple PCR reactions. Analysis of RNA-Seq data Three independent ESC lines were differentiated into EpiLCs for each genotype (male Kdm5c fl Y , Kdm5c Δ Y ; female Kdm5c fl/fl , Kdm5c Δ/Δ ). The EpiLCs were then homogenized in TRI Reagent BD (Sigma) and subjected to total RNA isolation using the RNEasy Mini Kit (Qiagen). Ribosomal RNA was depleted from total RNA using the RiboMinus Eukaryote Kit v2 for RNA-Seq (Life Technologies). Libraries were prepared using Direct Ligation of Adapters to First-strand cDNA as described previously [85] . Multiplexed libraries were pooled in approximately equimolar ratios and purified from a 1.8% TBE-agarose gel. Libraries were sequenced on the Illumina HiSeq2500 platform, with single-end 50 base pair reads, according to standard procedures. Detailed information on reverse transcription, adapter design, ligation, and subsequent steps has been described previously [85] . Raw reads were demultiplexed and filtered according to the standard Illumina analysis pipeline. Reads from sequencing libraries were mapped to the mm9 build of the mouse genome using Tophat 2 [86] , [87] (version 2.1.0), allowing up to one mismatch, and only uniquely mapped reads were analyzed further. Bigwig files normalized to the read depth were used to confirm the lack of reads from deleted KDM5C exons. Expression plasmids and lentiviral transduction in ESCs mKdm5c , hKDM5C , hKDM5D , oKdm5c , and oKdm5d were cloned from cDNAs into the Gateway Entry vector (pDONR221, Invitrogen). The pKdm5c cDNA sequence (Accession: XP_028923236) with the AttL1 and AttL2 recombination sequence at the 5´ and 3´ end, respectively was custom synthesized (Gene Universal Inc.). The hKDM5C(H514A) and oKdm5c(H514A) mutant cDNAs were generated by PCR-based mutagenesis. The sequence of all cDNAs was verified via Sanger sequencing. To generate the plasmids for stable overexpression in X ∆Tsix Y male ESCs, the cDNAs were cloned into an in-house generated PGK promoter-driven Strep-tag II lentiviral vector by Gateway LR recombination. To generate doxycycline-inducible constructs used for overexpression in XY male ESCs, the cDNAs were cloned into a PGK promoter-driven HA-tag lentiviral vector pLIX-402 (Addgene plasmid # 41394) by Gateway LR recombination. For the production of lentivirus, 50–70% confluent HEK293T cells in a 10-cm tissue culture plates were co-transfected with 3.33 μg lentiviral construct, 2.5 μg psPAX2 packaging plasmid, and 1 μg pMD2.G envelope plasmid using TransIT-293 (Mirus). Lentiviral particles were collected 48 h post transfection. The lentivral particles were then concentrated using LentiX (Clontech #631231). Concentrated lentivirus was transduced to ESCs with 10 μg/ml Polybrene (Millipore, #TR-1003-G). After 72 h, the transduced cells were selected with 3 μg/ml Puromycin (Sigma, #P8833-25MG) and subcloned to generate clonal cell lines. For inducible overexpression, cells were treated with 2 µg/ml doxycycline (Sigma) for 3 days. Media were changed every 24 h with fresh doxycycline. ChIP ChIP was performed as previously described [54] , with a minor modification, where we sonicated the chromatin using truChIP sonicator (Covaris). Two independent X ∆Tsix Y , X ∆Tsix;∆Kdm5c Y , or Tg-mKdm5c ; X ∆Tsix Y ESC lines were differentiated for 2 days (2d) beyond the epiblast-like cell (EpiLC) stage for ChIP with the exception that KDM5C ChIP was performed on one X ∆Tsix;∆Kdm5c Y 2d differentiated EpiLC sample. To achieve optimal inter-sample normalization of ChIP efficiency, Drosophila chromatin (Abcam #58083, 100 ng), which contains fly-specific histone variant H2Av, was spiked in and subsequently immunoprecipitated with 0.4 μg anti-H2Av antibody (Active Motif #39715) according to the manufacturer’s instructions. Two to five million EpiLCs were lysed and incubated with 3 μg of one of the following antibodies: H3K4me1 antibody (Abcam #8895); H3K4me2 antibody (Abcam #7766); H3K4me3 antibody (Abcam #8580); H3K27ac antibody (Active motif #39135); rabbit IgG antibody (Jackson Immuno Research #011-000-003); or 10 μg of an in-house anti-KDM5C antibody [54] . DNA was purified by phenol/chloroform extraction and eluted using QIAquick purification kit (QIAGEN#28104). ChIP-Seq ChIP-Seq libraries were sequenced on the Illumina HiSeq2500 platform to generate 50 bp single-end reads. Raw reads were demultiplexed and filtered according to the standard Illumina analysis pipeline. Reads from sequencing libraries were then mapped to the mouse (mm9) and fruit fly (dm6) genome assemblies using Bowtie [97] (version 1.2.2) allowing up to two mismatches. Only uniquely mapped reads were used for analysis. For KDM5C ChIP-Seq analysis, peaks were called using MACS2 software (version 2.1.0.20140616) [98] using input BAM files for normalization, with filters for a q -value <0.1 and a fold enrichment greater than 1. This analysis yielded 98 peaks on the X chromosome for d2 differentiated X ∆Tsix Y EpiLC samples; 1 peak for the X ∆Tsix;∆Kdm5c Y d2 EpiLC sample. For visualization in the Integrated Genome Viewer, reads were extended by 180 bp, and bigwig files were generated with coverage normalized using the number of mapped reads to the Drosophila genome (reads mapped per reference genome per million reads) [99] , [100] . ChIP-qPCR ChIP was performed as above. All qPCR reactions were performed using SYBR Green-based relative quantification method on an Eppendorf Realplex Mastercycler (software version 2.2.0.84). The following primers were used: Xist TSS downstream region (Region 1): forward CACAACCCCGCAAATGCTAC, reverse CGGCTATTCTCGAGCCAGTT; Xist promoter region (Region 2): forward ACTATGAGCGTAAGCCCACC, reverse CATGTATCGCTCCGCGTCTT; Xist upstream region (Region 3): forward GATCCATTCCATTAATACGAGCACT, reverse AGTTCACACTCCTCTGAGACCC. Fluorescent western blotting Protein lysates were made in RIPA buffer (50 mM Tris-HCl, 1% NP40, 0.25% Na-deoxycholate, 150 mM NaCl) with PMSF (Sigma, #P7626) and protease inhibitor cocktail (Roche, #11873580001). Lysates were mixed with Laemmli sample buffer and boiled for 10 min prior to loading on polyacrylamide gels. Resolved proteins were transferred onto PVDF membranes (iBlot 2 PVDF, Invitrogen #IB24002) following the manual instructions for 7 min (iBlot 2 Dry Blotting System, Invitrogen #IB21001). Membranes were then blocked by Intercept Blocking Buffer (LI-COR, #927-70001) for 1 h at room temperature and incubated in the anti-Strep-Tag II (GenScript, #A01732-100; 1:1000 dilution) and anti-KDM5C (Abcam, #194288; 1:1000 dilution) primary antibodies together overnight at 4 °C. Appropriate Li-COR IRDye series (680LT, #926-68020/800CW, #926-32211) secondary antibodies were used (1:20,000 dilution). Blots were scanned using the Odyssey CLx Imager (Li-COR Biosciences) following the manufacturer’s instructions. Results were analyzed using Image Studio (Version 5.2). Transgenic proteins levels were normalized to KDM5C. Microscopy Images of all stained samples were captured using a Nikon Eclipse TiE inverted microscope with a Photometrics CCD camera. The images were analyzed after deconvolution using NIS-Elements software (version 5.20.02, Build 1453). All images were processed uniformly. KDM5C/KDM5D sequence analysis Amino acid sequences were obtained from the Ensembl database and from Cortez et al., 2014 [7] . Human KDM5C accession NP_004178 human KDM5D accession NP_001140177 mouse KDM5C accession XP_006528832 mouse KDM5D accession NP_035549 elephant KDM5C ensemble transcript ID ENSLAFT00000027692.1 ( https://useast.ensembl.org/Loxodonta_africana/Transcript/Summary?db=core;g=ENSLAFG00000000303;r=scaffold_85:1408730-1440791;t=ENSLAFT00000027692 ), elephant KDM5D accession JAC06693 opossum KDM5C accession GAQH01000002 opossum KDM5D accession JAC06620 platypus KDM5C accession XP_028923236 and chicken KDM5A accession XP_416379 Multiple sequence alignment was performed using ClustalW [77] (version 2.1). MSAViewer [101] (version 1.12.0) tree tool was used to create a rooted phylogenetic tree with branch lengths according to the Neighbor-Joining algorithm. Amino acid positions for the JmjC domains were acquired from the NCBI Conserved Domain Database [102] . Iron and α-ketoglutarate-binding sites were acquired from UniProt for human KDM5C and the human amino acid positions were compared to the other species [55] , [76] , [103] . Analysis of Kdm5c expression in therian and platypus females vs. males Raw RNA-Seq fastq files were obtained from the NCBI Sequence Read Archive. RNA-seq data for human, chimp, bonobo, macaque, mouse, opossum, and platypus are available under GEO accession number GSE30352 [71] . RNA-seq data for rat and marmoset are available under GEO accession number GSE50747 [7] , [104] . Echidna RNA-seq data is available under project accession number PRJNA591380 [73] . The brain and cerebellum data were combined into one “brain” sample. One male and one female sample of each brain, heart, kidney, and liver were processed in each species. The human dataset did not include a female liver sample, and so the liver was left out of the human analysis. Reads were mapped to the latest assembly reference genome for a given species using STAR (v2.5.2a), and reads were counted using HTseq (Python v2.7). Genes in a sample were only included in the analysis if they contained at least 10x read coverage. A gene was included if at least one tissue type met these criteria in male and female samples. For Kdm5c expression plots, Kdm5c TPM (transcripts per kilobase per million RNA-Seq reads) was calculated in each tissue (brain, heart, kidney, and liver), and TPM values for each tissue were plotted. For average X chromosome plots (or Chromosome 6 for platypus and echidna), TPM values of all genes were averaged in each tissue. Average TPM values for each of the four tissues were plotted. For dot plots, the TPM values from each tissue were averaged for each gene. Tissue averages for each gene were used to calculate Log2 fold change between females and males and plotted against the gene’s chromosome position. Gene length, for TPM calculations, was acquired from the RefSeq annotation for each species. Statistical analysis could not be performed due to a lack of biological replicates. See Supplemental Tables 6 – 17 . Statistical analysis Welch’s two-sided t test was performed using Microsoft Excel. Chi-square analysis of RNA FISH was performed using R (version 4.1.2). All exact P values are provided in Supplementary Tables 1 – 9 . Reporting summary Further information on research design is available in the Nature Research Reporting Summary linked to this article.